Genome-wide deserts for copy number variation in vertebrates Most copy number variations are neutral, but some are deleterious and associated with various human diseases. Copy number variations are distributed non-randomly in vertebrate genomes, and it was recently reported that ohnologs, which are duplicated genes derived from whole genome duplication, are refractory to copy number variations. However, it is unclear what genomic factors affect the deleterious effects of copy number variations and the biological significance of the biased genomic distribution of copy number variations remains poorly understood. Here we show that non-ohnologs neighbouring ohnologs are unlikely to have copy number variations, resulting in ohnolog-rich regions in vertebrate genomes being copy number variation deserts. Our results suggest that the genomic location of ohnologs is a determining factor in the retention of copy number variations and that the dosage-balanced ohnologs are likely to cause the deleterious effects of copy number variations in these regions. We propose that investigating copy number variation of genes in regions that are typically copy number variation deserts is an efficient means to find disease-related copy number variations. Gene duplication is a frequent occurrence in eukaryotic genomes, with most duplicated genes being generated by intrachromosomal tandem duplication events and through retrotransposition events [1] . Ongoing gene duplication or loss results in polymorphism at the population level, and these copy number variations (CNVs) have been observed in many organisms [2] , [3] , [4] , [5] , [6] , [7] , [8] , [9] . CNVs are frequently associated with human disease, and therefore it is important to understand the factors that influence the generation of CNVs in a genome [10] , [11] , [12] , [13] , [14] , [15] . CNVs are not randomly distributed in eukaryotic genomes, in particular they tend to be located close to telomeres and centromeres [5] , [16] . It has been reported that non-homologous end-joining, transposable elements [17] and DNA replication time [18] , [19] are also associated with CNVs. Segmental duplications (SDs) strongly correlate with CNVs [20] , and it has been proposed that SDs induce recurrent duplications through non-allelic homologous recombination resulting in the generation of CNV hotspots [9] , [21] . Whole genome duplication (WGD) occurred early in the vertebrate lineage [22] , [23] , [24] . Duplicated genes derived from WGD (ohnologs) are refractory to CNVs and small-scale duplication (SSD) [25] , probably due to dosage balance constraints [26] , [27] , [28] , [29] . Dosage balance may exist between dosage-sensitive genes participating in the same biological process, especially genes contributing peptides to the same protein complex [30] , [31] , [32] , [33] , [34] . Change in the relative amounts of dosage-balanced genes (DBGs) is deleterious, and the expectation is that duplication of these genes will not be tolerated except when the duplication is itself balanced. WGD duplicates all genes simultaneously and therefore does not perturb relative dosages [35] . The deleterious effects of CNV of a DBG are predictable, however, the broader significance and the incidental effects of dosage-constrained genes on the evolution of neighbouring genes remain poorly understood. CNVs often include more than one gene. In fact, over 90% (6,055/6,711) of genes within CNVs in the Database of Genomic Variants ( http://projects.tcag.ca/variation ) were within CNVs that include multiple genes. CNV events can occur anywhere in the genome, although the CNV mutation rate varies across the genome. Notwithstanding other factors that influence CNV frequency, we predict that duplication of a genomic fragment including a DBG such as an ohnolog will be deleterious, resulting in their removal from the population. According to this idea, even non-DBGs on a genomic fragment including an ohnolog are unlikely to duplicate. Therefore, we hypothesize that genomic regions neighbouring ohnologs are CNV deserts due to the incidental effects of the presence of dosage-constrained genes. We find non-ohnologs neighbouring ohnologs are unlikely to display CNVs, and observe CNV deserts in ohnolog-rich regions (ORRs). Similarly, probable dosage-sensitive singletons that are unduplicated in all vertebrate lineages also repress CNVs of their immediate neighbours. In addition, long CNVs, prone to overlap genes, are less frequently observed near ohnologs. We predict that, by contrast, generation of CNVs is a predominantly neutral event outside ORRs. Consistent with this, we show that olfactory receptor genes, which constitute the largest multigene family and thus have experienced evolutionary CNV, are less likely to be located in ORRs. Our findings provide a new important insight into the genomic factors affecting the fitness effects of CNVs and gene duplications. Less frequent CNVs of genes neighbouring ohnologs To investigate whether the proportion of genes displaying CNV ( P CNV ) for non-ohnologs neighbouring ohnologs is low, we estimated distances between non-ohnologs and their closest ohnolog ( Supplementary Data 1 ). We found a strong positive correlation between P CNV and distance to ohnologs for non-ohnologous genes on a 0.0–2.0Mb scale ( Fig. 1a ; R =0.98, P =1.4 × 10 −7 , product-moment correlation coefficient). This indicates that genomic regions near ohnologs are resistant to CNVs. Strikingly, more than 80% of non-ohnologs located>1.5 Mb from the closest ohnolog displayed CNVs ( Fig. 1a ), although 30% (48/160) of them are on the Y chromosome. Note that we observed a significant correlation even after removal of Y chromosome genes ( R =0.98, P =2.6 × 10 −7 , product-moment correlation coefficient). We observed a similar trend over shorter genomic regions ( Supplementary Fig. S1 ; 0.0–0.5 Mb: R =0.78, P =0.0044 and 0.0–1.0 Mb: R =0.89, P =0.00026, product-moment correlation coefficient). In order to verify that this effect is not a consequence of low-quality CNV detection, we also examined the relationship between the proportion of genes with validated CNVs from Conrad et al. [36] and distance to ohnologs for non-ohnologous genes. This data set does not include any Y chromosome CNVs, so we excluded Y chromosome genes from this analysis. We found a significant positive correlation between P CNV and distance to ohnologs for non-ohnologous genes on a 0.0–0.5 Mb scale ( Fig. 2a ; R =0.87, P =0.00058, product-moment correlation coefficient), 0.0–1.0 Mb scale ( Fig. 2b ; R =0.88, P =0.00030, product-moment correlation coefficient) and 0.0–2.0 Mb scale ( Fig. 2c ; R =0.70, P =0.017, product-moment correlation coefficient). This result supports our hypothesis even with this more stringent CNV data set. 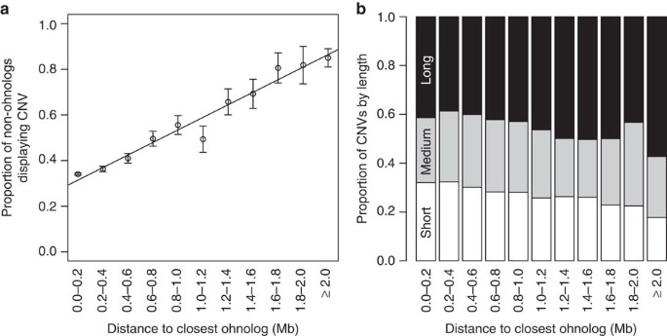Figure 1: Relationship between CNVs and distance to closest ohnolog. (a) Relationship between the proportion of non-ohnologs with CNV and distance to their closest ohnolog for non-ohnologs. Y axis indicates the proportion of non-ohnologs with CNVs for each distance. Error bars represent s.e. (b) Relationship between CNVs and the distance to their closest ohnolog for all CNVs. CNVs are classified into three categories (white: short, grey: medium and black: long) based on their length. Y axis indicates that proportion of CNVs by length for each fraction. Figure 1: Relationship between CNVs and distance to closest ohnolog. ( a ) Relationship between the proportion of non-ohnologs with CNV and distance to their closest ohnolog for non-ohnologs. Y axis indicates the proportion of non-ohnologs with CNVs for each distance. Error bars represent s.e. ( b ) Relationship between CNVs and the distance to their closest ohnolog for all CNVs. CNVs are classified into three categories (white: short, grey: medium and black: long) based on their length. Y axis indicates that proportion of CNVs by length for each fraction. 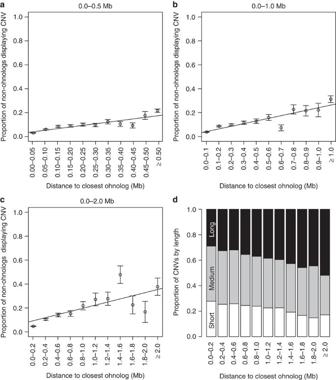Figure 2: Relationship between validated CNVs and distance to closest ohnolog. (a–c) Y axis indicates the proportion of genes having CNVs for each distance class. Error bars represent s.e. Relationship between genes with validated CNV from ref36and distance to their closest ohnologs for non-ohnologs (a: 0.0–0.5 Mb,b: 0.0–1.0 Mb andc: 0.0–2.0 Mb). (d) Relationship between validated CNVs from ref36and distance to their closest ohnolog for all CNVs. CNVs are classified into three categories (white: short, grey: medium and black: long) based on their length. Y axis indicates that proportion of CNVs by length for each fraction. Full size image Figure 2: Relationship between validated CNVs and distance to closest ohnolog. ( a – c ) Y axis indicates the proportion of genes having CNVs for each distance class. Error bars represent s.e. Relationship between genes with validated CNV from ref 36 and distance to their closest ohnologs for non-ohnologs ( a : 0.0–0.5 Mb, b : 0.0–1.0 Mb and c : 0.0–2.0 Mb). ( d ) Relationship between validated CNVs from ref 36 and distance to their closest ohnolog for all CNVs. CNVs are classified into three categories (white: short, grey: medium and black: long) based on their length. Y axis indicates that proportion of CNVs by length for each fraction. Full size image Some singletons may also be dosage sensitive. We identified putative dosage-sensitive singletons as genes present in single copy in all of human, chimpanzee, macaque, mouse, rat, dog, cow, opossum and chicken. We examined CNVs neighbouring these 1,151 singletons and found that they were unlikely to display CNVs (21.9%, 252/1,151; P =3.0 × 10 −14 , χ 2 test), which is consistent with the hypothesis that these are dosage-sensitive genes [37] . We observed a strong positive correlation between P CNV of non-singletons and distance to singletons for non-singletons on a 0.0–0.5 Mb scale ( Supplementary Fig. S1 ; R =0.94, P =1.36 × 10 −5 , product-moment correlation coefficient). This consistently indicates that dosage-sensitive genes affect CNVs of neighbouring genes. On the other hand, there was no significant correlation on larger scales ( Supplementary Fig. S1 ; 0.0–1.0 Mb and 0.0–2.0 Mb). There are many ohnologs (7,294) compared with dosage-sensitive singletons (1,151) in the human genome, which means that long genomic intervals without any singletons are unlikely to also be without any ohnolog, and the effect of the presence of an ohnolog may hinder our ability to detect a relationship between proximity to a singleton and CNVs over longer scales, even if that relationship is present. Recently, Springer et al. [38] reported that syntenic genes between rice and maize were unlikely to display CNVs. Ohnologs often remain in synteny (paralogons) [23] , [39] , and we speculated that the enrichment of conserved synteny within the ohnolog gene set might affect the above results. Therefore, we examined the relationship between P CNV and syntenic genes (human–chicken). There was no significant correlation between P CNV and distance to the closest syntenic genes for non-syntenic genes in larger scales ( Supplementary Fig. S1 ; 0.0–1.0 Mb and 0.0–2.0 Mb), although there was a weak correlation only in 0.0–0.5 Mb scale ( Supplementary Fig. S1 ; R =0.67, P =0.023, product-moment correlation coefficient). Although syntenic genes were unlikely to display CNVs themselves (23.3%, 2,562/10,979; P <2.2 × 10 −16 , χ 2 test), gene synteny could be maintained by random chance under neutral selection or other factors regardless of dosage sensitivity. Therefore, the influence of syntenic genes on CNV of neighbouring genes is weaker than that of ohnologs. If our hypothesis is correct, short CNVs should occur near ohnologs more frequently than long CNVs, because long CNVs have a greater chance to contain multiple genes including an ohnolog ( Fig. 3 ). We classified CNVs in three categories, which are short (<3 kb), medium (3–10 kb) and long CNVs (≥10 kb), and estimated their distance to the closest ohnolog. We found that long CNVs were unlikely to be observed near ohnologs compared with short CNVs ( Fig. 1b ; P =3.9 × 10 –5 , Mann–Whitney U test). We observed the same trend using validated CNVs from Conrad et al. [36] and ( Fig. 2d ; P <2.2 × 10 −16 , Mann–Whitney U test). These results indicate that the resistance of ohnologs to duplication/deletion also influences duplication/deletion of neighbouring regions in a way that is proportional to the distance from the ohnolog. 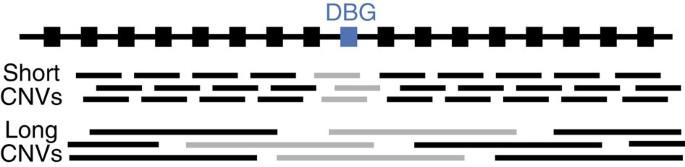Figure 3: Hypothetical relationship between the length of the deleterious CNVs and DBGs. Boxes, horizontal lines and partial lines indicate genes, genomes and CNVs, respectively. Blue and black boxes are DBGs (such as ohnologs) and others, respectively. Partial grey lines indicate deleterious CNVs including DBGs. The longer a CNV is, the more frequently the CNV contains DBGs. Therefore, near ohnologs, short CNVs are more likely to be benign than long CNVs. Figure 3: Hypothetical relationship between the length of the deleterious CNVs and DBGs. Boxes, horizontal lines and partial lines indicate genes, genomes and CNVs, respectively. Blue and black boxes are DBGs (such as ohnologs) and others, respectively. Partial grey lines indicate deleterious CNVs including DBGs. The longer a CNV is, the more frequently the CNV contains DBGs. Therefore, near ohnologs, short CNVs are more likely to be benign than long CNVs. Full size image Ohnolog-rich regions To test for a genome-wide tendency of resistance to CNVs caused by the presence of ohnologs, we conducted a sliding window analysis (2 Mb window and 0.2 Mb sliding). We defined human genomic regions with the proportion of ohnologs ( P ohno )≥50% in a 2 Mb window as (ORRs; Supplementary Data 2 ). We found that non-ohnolog genes with CNVs were unlikely to overlap ORRs and furthermore, the peaks of P CNV were rarely in ORRs ( Fig. 4 and Supplementary Fig. S2a ). In fact, there was a significant negative correlation between the P ohno and P CNV for 2 Mb windows ( R =−0.25, P <2.2 × 10 −16 , product-moment correlation coefficient). Note that we only used windows including non-ohnologs for estimating the correlation coefficient. Even when we used non-overlapping windows (2 Mb window and 2 Mb sliding), we observed the same trend ( R =−0.26, P <2.2 × 10 −16 , product-moment correlation coefficient). Furthermore, we observed that there was a significant negative correlation between P ohno and P CNV for 2 Mb windows using validated CNVs from Conrad et al. [36] ( R =−0.22, P <2.2 × 10 −16 , product-moment correlation coefficient). These results indicate that we successfully observe ‘CNV deserts’ due to the enrichment of ohnologs even on a genome-wide level. We also observed that there was a significant negative correlation between P ohno and P CNV for different window sizes (0.5 Mb: R =−0.10, P <2.2 × 10 −16 ; 1 Mb: R =−0.16, P <2.2 × 10 −16 ; 4 Mb: R =−0.34, P <2.2 × 10 −16 and 8 Mb: R =−0.41, P <2.2 × 10 −16 ). Although the fine-scale landscape of ORRs would be much more informative for understanding the relationship between the proximity of DBGs and CNVs, the average number of genes per window for short window sizes was small (0.5 Mb window: 3.8 genes and 1 Mb window: 7.1 genes) resulting in large variation in both P ohno and P CNV compared with longer window sizes (2 Mb window: 13.8 genes, 4 Mb window: 27.0 genes and 8 Mb window: 52.9 genes). Therefore, we chose the 2-Mb window size for the following analyses. 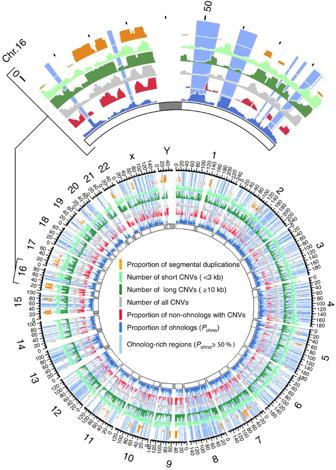Figure 4: Distributions of CNVs and ohnologs in a human genome. A sliding window analysis was conducted (window size: 2 Mb). This figure shows human chromosomes including several CNV patterns. Grey boxes indicate centromere or telomere. Blue lines represent the proportion of ohnologsPohnofor each window. Light blue lines indicate ORRs where thePohnois≥50%. Red lines represent the proportion of non-ohnologs having CNV. Grey, green and light green lines represent the number of all CNVs (max: 100), long CNVs (≥10 kb; max:30) and short CNVs (<3 kb; max:30) for each window, respectively. Orange lines denote the proportion of intrachromosomal SDs (>5 Kb and>90% identity) from Human Genome Segmental Duplication Database44per 2-Mb window. This figure was made by CIRCOS (http://circos.ca). Blown-up chromosome 16 is shown in this figure as a typical example. Figure 4: Distributions of CNVs and ohnologs in a human genome. A sliding window analysis was conducted (window size: 2 Mb). This figure shows human chromosomes including several CNV patterns. Grey boxes indicate centromere or telomere. Blue lines represent the proportion of ohnologs P ohno for each window. Light blue lines indicate ORRs where the P ohno is≥50%. Red lines represent the proportion of non-ohnologs having CNV. Grey, green and light green lines represent the number of all CNVs (max: 100), long CNVs (≥10 kb; max:30) and short CNVs (<3 kb; max:30) for each window, respectively. Orange lines denote the proportion of intrachromosomal SDs (>5 Kb and>90% identity) from Human Genome Segmental Duplication Database [44] per 2-Mb window. This figure was made by CIRCOS ( http://circos.ca ). Blown-up chromosome 16 is shown in this figure as a typical example. Full size image To further test our hypothesis, we compared the allele frequency of CNVs within ORRs with that outside ORRs. We obtained allele frequencies for 7,305 validated deletions that were larger than 1 kb from the 1,000 Genomes Project [40] . Genomic locations for the deletions based on human genome assembly hg19 were converted to those based on hg18 by liftOver ( http://genome.ucsc.edu/cgi-bin/hgLiftOver ). We observed that the allele frequency of deletions overlapping ORRs (average: 4.4%) was significantly lower than those outside ORRs (average: 5.0%; P =1.3 × 10 −7 , Mann–Whitney U test). This result consistently indicates that CNVs are unlikely to occur within ORRs. Gene density varies across the human genome, and the biased gene distribution may affect the above window analysis [20] . In fact, windows with higher gene density also have higher P CNV of non-ohnologs ( Fig. 5 ). To correct for this potential bias, we classified windows into seven bins according to their gene density (number of genes per Mb), and compared P CNV of non-ohnologs inside ORRs and outside ORRs, using the same gene density bins. We found that P CNV of non-ohnologs within ORRs was lower than those outside ORRs with any gene density ( Fig. 5 ). 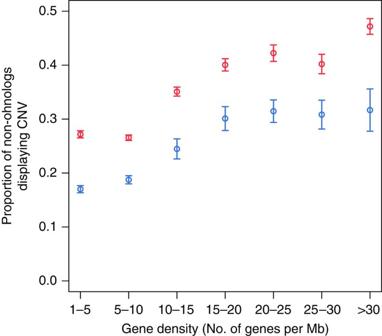Figure 5: Proportion of non-ohnologs with CNVs under different gene density. X axis indicates the number of genes per Mb in a window. Y axis indicates the proportion of non-ohnologs having CNVs (PCNV). Blue and red circles denotePCNVin ORRs and that outside ORRs in 2-Mb windows of the human genome, respectively. The number of windows in ORRs and outside ORRs are 3,954 and 9,239, respectively. Error bars represent s.e. Figure 5: Proportion of non-ohnologs with CNVs under different gene density. X axis indicates the number of genes per Mb in a window. Y axis indicates the proportion of non-ohnologs having CNVs ( P CNV ). Blue and red circles denote P CNV in ORRs and that outside ORRs in 2-Mb windows of the human genome, respectively. The number of windows in ORRs and outside ORRs are 3,954 and 9,239, respectively. Error bars represent s.e. Full size image As shown above, long CNVs are more likely to be observed far from ohnologs compared with short CNVs ( Fig. 1b ). We examined the distributions of short and long CNVs in ORRs. Long CNV were significantly located outside ORRs ( Fig. 4 and Supplementary Fig. S2b ; P =0.00090, χ 2 test). On the other hand, short CNVs tended to have an even distribution in the human genome except for genomic regions close to telomeres and centromeres [5] , [16] , ( Fig. 4 and Supplementary Fig. S2c ). This observation is consistent with our hypothesis ( Fig. 3 ). Moreover, long CNVs were found to be enriched in cases as compared with controls for various congenital defects [41] . The probability of the disruption of genomic function through CNVs must be higher for long CNVs than for short CNVs. The difference in the deleterious effect between long and short CNVs would be particularly prominent within the dosage-sensitive regions. We propose that long CNVs are frequently subject to selective constraints, whereas short CNVs are primarily influenced by the mutation rate. We classified CNVs into intergenic or intragenic CNVs, and investigated their frequencies within or outside ORRs. Intragenic long CNVs were significantly enriched in genomic regions outside ORRs (62.9%, 8676/13,801) compared with intragenic short CNVs (49.0%, 3,437/7,012; P <2.2 × 10 −16 , χ 2 test). On the other hand, there was no significant difference in the frequency of intergenic long CNVs outside ORRs (41.1%, 4,375/10,665) compared with that of intergenic short CNVs outside ORRs (40.1%, 4,444/11,090). This result indicates that long CNVs including genes are unlikely to occur within ORRs. Furthermore, we observed that CNVs in seven other vertebrate species reported by different research groups (chimpanzee [8] , macaque [7] , mouse [6] , rat [5] , dog [4] , cow [3] and chicken [2] ) were unlikely to overlap ORRs in those genomes ( Supplementary Fig. S3a–g ; chimpanzee: R =−0.10, P <2.2 × 10 −16 ; macaque: R =−0.07, P =4.1 × 10 −15 ; mouse: R =−0.25, P <2.2 × 10 −16 ; rat: R =−0.12, P <2.2 × 10 −16 ; dog: R =−0.14, P <2.2 × 10 −16 ; cow: R =−0.12, P <2.2 × 10 −16 and chicken: R =−0.067, P =1.8 × 10 −6 , product-moment correlation coefficient). As ohnologs tend to be conserved across genomes and in conserved synteny, this observation is consistent with observations that CNV hotspots are shared between human and chimpanzee genomes [8] , [9] and between mouse and rat [5] , and supports our hypothesis of a consistent deleterious effect of duplication of ORRs. Dosage sensitivity of non-ohnologs within ORRs About 40% (8,240/20,907) of human genes (4,321 ohnologs and 3,919 non-ohnologs) were in ORRs. We found that P CNV of non-ohnologs was significantly lower in ORRs (24.2%) than elsewhere in the genome (40.7%, P <2.2 × 10 −16 , χ 2 test), and that P CNV of ohnologs was significantly lower in ORRs (19.5%) than in the remainder of the genome (32.7%, P <2.2 × 10 −16 , χ 2 test; Table 1 ). Interestingly, P CNV of ohnologs outside ORRs (32.7%) was significantly higher than that of non-ohnologs in ORRs (24.2% P =6.4 × 10 −15 , χ 2 test). Not all ohnologs are expected to be dosage-balanced, so ORRs have a greater chance of including a true-positive dosage-balanced ohnolog. There may also be an effect of the combined burden of simultaneous duplication or loss of multiple dosage-balanced ohnologs within a single CNV and this is more likely within ORRs due to physical clustering. Table 1 Difference in properties between genes within and outside ohnolog-rich regions. Full size table It has been reported that protein complex genes are often DBGs [35] . We found that non-ohnologous protein complex genes were significantly enriched in ORRs compared with non-ohnologs outside ORRs ( Table 1 ; P =2.6 × 10 –9 , χ 2 test). Furthermore, non-ohnologs within ORRs were likely to be singletons in all genomes analysed (purported dosage-sensitive singletons as described above; Table 1 ; P =1.0 × 10 –8 , χ 2 test). The dosage-sensitive singletons within ORRs are likely to be genes that returned to single-copy status from ohnologs after WGD [37] . These results indicate that non-ohnologs within ORRs may also be dosage-sensitive genes. Previously reported candidate genes for diseases associated with pathogenic CNVs are frequently ohnologs [25] . Notably, non-ohnologs in ORRs were also significantly enriched in disease genes ( Table 1 ; P =4.1 × 10 –5 , χ 2 test). Other genomic factors influencing CNVs SDs are evolutionarily fixed duplications that arise through non-allelic homologous recombination mechanisms and that prior to fixation exist as a major class of CNVs [20] . Consistent with this, we observed a strong correlation between SDs and CNVs ( R =0.27, P <2.2 × 10 −16 , product-moment correlation coefficient). SDs are clearly a significant causal factor in CNV hotspots. Other factors have also been linked to CNV and gene duplication frequency [20] . We considered whether these alternative genomic elements might explain CNV deserts better than ORRs. CNVs are rarely observed in ultraconserved elements [42] or in methylation deserts [43] , but these constitute a small portion of the genome, and do not explain genome-wide trends. CNVs tend to be close to telomeres and centromeres [5] , [16] , [17] , [20] , a trend that was also observed for 2 Mb windows in our study ( R =−0.25, P <2.2 × 10 −16 , product-moment correlation coefficient). However, this is not informative about the distributions of CNVs in the rest of the genome. It has been also reported that Alu , processed pseudogenes, recombination rate and gene density are associated with CNVs [2] , [17] , [20] , [36] . We employed a multiple regression model in which P CNV of non-ohnologs and the number of CNVs (all, short, or long CNVs) were used as objective variables and P ohno , the number of Alu , the number of processed pseudogenes, the number of genes and the average recombination rates were used as explanatory variables for 2 Mb windows in the human genome. Genomic locations of Alu and processed pseudogenes were obtained from Ensembl database (release 52). We downloaded fine-scale recombination rates generated by the HapMap project ( http://hapmap.ncbi.nlm.nih.gov ) and estimated average recombination rates for each 2 Mb window. As reported in previous studies, all factors were significantly associated with the number of CNVs ( Table 2 ). Particularly, P ohno was the strongest factor for explaining P CNV and the number of long CNVs, although P ohno was a significant factor but not the strongest one for explaining the number of all or short CNVs. This is consistent with our hypothesis and the above result ( Figs 1b , 3 and Supplementary Fig. S2 ). To rigorously avoid any potential error coming from the analysis strategy, we also compared ohnologs and CNVs ( P CNV and the number of long CNVs) using non-overlapping 2 Mb windows. The results are consistent and the P- values are even more convincing ( Supplementary Table S1 ). These results indicate that ORRs are one of the most important factors influencing CNVs of genes at a genome-wide level. Table 2 Multiple regression analysis indicating the relationship between CNVs and their candidate causal factors. Full size table SD hotspots without CNVs are likely to overlap ORRs SDs are thought to induce genomic rearrangements if they are closely located and in direct orientation, thus resulting in the enrichment of CNVs in the region. [9] , [20] , [21] . A recent study reported 111 SD hotspots mediated by non-allelic homologous recombination, and the authors investigated the presence of CNVs in the hotspots [41] . The frequency of CNVs in SD hotspots is elevated in genomic regions where the SDs are in direct orientation (85.2%, 46/54) compared with those with SDs in inverted orientation (28.1%, 16/57) [41] . However, the high frequency of CNVs might ensure a steady supply of SDs in direct orientation. Namely, it is unclear whether SDs in direct orientation cause CNVs or the frequent CNVs continue to produce SDs in direct orientation during evolution. We propose that ORRs are an important repressor of CNVs. If the presence of closely located SDs in direct orientation is an important factor causing frequent CNVs, SD hotspots with CNVs should be frequently observed in genomic regions with direct SDs repeats regardless of their overlapping ORRs. Therefore, we examined the frequency of overlap with ORRs for the SD hotspots. Note that the designation of inactive SD hotspots indicates that no CNVs were observed in the region in healthy individuals. Out of 49 inactive SD hotspots (that is, without CNVs), 31 overlap with ORRs (63%). The proportion of inactive hotspots with ORR overlaps was consistent for both direct and indirect SDs ( Supplementary Table S2 ; 5/8 direct SDs and 26/41 indirect SDs). We also found a low frequency of overlap with ORRs for active SD hotspots (with CNVs) regardless of SD orientation (direct orientation: 30.4%, 14/46; inverted orientation: 31.3%, 5/16; Supplementary Table S2 ). We speculate that these inactive hotspots appear to be inactive due to the purifying selection on CNVs of dosage-sensitive genes such as ohnologs. To estimate the expected proportion of SD hotspots overlapping ORRs, we shuffled the genomic location of the hotspots randomly 1,000 times. Note that we excluded chromosome Y, telomeres and centromeres for the shuffling, because there were no SD hotspots in those regions. We observed that SD hotspots were significantly more likely to be located outside ORRs (observation: 45.0% versus expectation: 74.9%, P =7.9 × 10 −14 , Z -test). When we also consider the combination of CNVs and SD hotspots, we observe that the effect is even stronger, with SD hotspots that also have CNVs being severely depleted in ORRs (observation: 30.6% versus expectation: 74.8%; Z-score=−7.84, P =4.4 × 10 −15 , Z -test) compared with SD hotspots not having any CNVs (observation: 63.2% versus expectation: 75.4%; Z -score=−2.06, P =0.039, Z -test). This consistently indicates that genomic locations displaying CNVs are unlikely to overlap with ORRs. SSD deserts SSD genes arise initially as CNVs in a population. Consistent with this, we found a significant trend that SSD genes are unlikely to neighbour ohnologs ( R =0.81, P =0.0027, product-moment correlation coefficient). We also observed that segmental duplications [44] had a strong tendency to be located outside ORRs (observation: 22.5% versus expectation: 60.4%; Z -score=−76.0, P =0, Z -test; Fig. 4 ). As mentioned above, ORRs tend to be conserved across vertebrates, thus we predict that human genes in ORRs and their vertebrate orthologs should have rarely experienced SSD during evolution. To test this hypothesis, we obtained orthologs (one-to-one, one-to-many and many-to-many) between human and eight vertebrates (chimpanzee, macaque, mouse, rat, dog, cow, opossum and chicken) from the Ensembl database, and mapped SSD events on the human genome ( Fig. 6 ). Non-ohnologous genes without SSD in both human and vertebrate lineages frequently overlap human ORRs ( Fig. 6 ). In fact, there was a statistically significant correlation between the proportion of non-ohnologous genes without SSD and P ohno for 2 Mb non-overlapping windows (chimpanzee: R =0.30, P <2.2 × 10 −16 ; macaque: R =0.29, P <2.2 × 10 −16 ; mouse: R =0.26, P <2.2 × 10 −16 ; rat: R =0.26, P <2.2 × 10 −16 ; dog: R =0.27, P <2.2 × 10 −16 ; cow: R =0.29, P <2.2 × 10 −16 ; opossum: R =0.23; P <2.2 × 10 −16 and chicken: R =0.22, P =4.4 × 10 −16 , product-moment correlation coefficient), while SSD frequently occurred outside ORRs. This is consistent with our prediction that ORRs are SSD deserts across all vertebrate genomes and that the presence of ohnologs influences copy number changes during evolution. These observations clearly show the difference in the evolutionary gene duplication pattern between genes inside and outside ORRs. 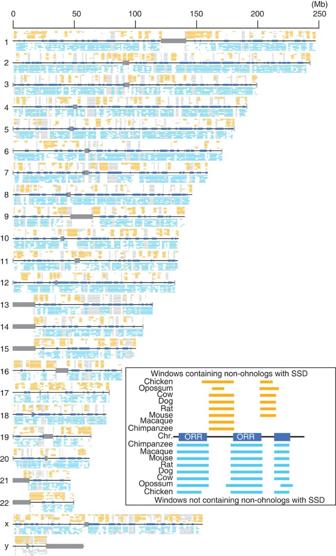Figure 6: Small-scale gene duplication deserts in humans. Horizontal black lines indicate human chromosomes with each chromosome number. Grey boxes on a chromosome indicate centromere or telomere. Sliding window analysis was conducted (window size: 2 Mb), and the proportion of ohnologs (Pohno) was estimated for each window. Blue lines indicate ORRs where thePohnois≥50% for each window. Orange lines over each chromosome shows windows in which there is at least one SSD in human lineage after speciation from a common ancestor of a compared vertebrate species (chimpanzee, macaque, mouse, rat, dog, cow, opossum and chicken from bottom) for non-ohnologs. Light blue lines under each chromosome show windows in which there are no SSDs for orthologous gene pairs between human and a compared vertebrate species (chimpanzee, macaque, mouse, rat, dog, cow, opossum and chicken from top) for non-ohnologs. If there are no orthologs for non-ohnologs in a window, the window was indicated in grey. Figure 6: Small-scale gene duplication deserts in humans. Horizontal black lines indicate human chromosomes with each chromosome number. Grey boxes on a chromosome indicate centromere or telomere. Sliding window analysis was conducted (window size: 2 Mb), and the proportion of ohnologs ( P ohno ) was estimated for each window. Blue lines indicate ORRs where the P ohno is≥50% for each window. Orange lines over each chromosome shows windows in which there is at least one SSD in human lineage after speciation from a common ancestor of a compared vertebrate species (chimpanzee, macaque, mouse, rat, dog, cow, opossum and chicken from bottom) for non-ohnologs. Light blue lines under each chromosome show windows in which there are no SSDs for orthologous gene pairs between human and a compared vertebrate species (chimpanzee, macaque, mouse, rat, dog, cow, opossum and chicken from top) for non-ohnologs. If there are no orthologs for non-ohnologs in a window, the window was indicated in grey. Full size image Olfactory receptor genes have expanded in the tetrapod lineage by massive gene duplications and formed one of the largest multigene families [45] . Olfactory receptors are important for detecting signals from the environment. Detecting thousands of different chemicals in the environment is essential for many organisms, and about 4% of vertebrate genes encode proteins related to smell [46] . It has been shown that olfactory receptor genes are located non-randomly in the genome [45] with clustering of those having similar functions. These gene clusters were probably created by tandem gene duplications. In addition, it is known that olfactory receptor genes often display CNVs [45] . We speculated that the biased gene distribution of the largest gene family may have been influenced by ORRs. We examined the genomic distribution of 442 and 1,111 olfactory receptor genes in human [47] and mouse [48] , respectively. Note that we defined human genomic regions with the number of ohnologs per non-olfactory receptor genes≥50% in a 2-Mb window as ORRs for this analysis. We observed that most olfactory receptor genes were located outside ORRs both for human ( Supplementary Fig. S4a ) and mouse ( Supplementary Fig. S4b ). Interestingly, not only genomic regions with a high density of olfactory receptor genes but also those with a low density of the genes were located outside ORRs ( Supplementary Fig. S4a,b ). We suggest that the genomic location of genes may facilitate the successful expansion of gene families such as the olfactory receptor genes. We demonstrate that genomic regions containing ohnologs have low duplicability, resulting in CNV deserts. Undoubtedly, SDs correlate with CNVs, however the mechanism to generate CNV hotspots by recurrent duplications through SDs is just one of the important direct factors influencing CNV distributions [9] , [21] . Our observations suggest that the genomic location of ohnologs, which are frequently DBGs, is an additional significant factor in the generation of the biased distribution of CNVs in vertebrate genomes. In particular, we show that the resistance to CNVs for genomic regions near ohnologs has a profound effect on long CNVs ( Fig. 1b , Supplementary Fig. S2b and Table 2 ). For the same reasons of dosage balance, ORRs are SSD deserts in vertebrate genomes. Conversely, CNV/SSD hotspots are located in ohnolog-poor regions where CNV is less likely to be deleterious, and result in the expansion of multi gene families such as the olfactory receptor gene family. Furthermore, we observe that non-ohnologs within ORRs are likely to be dosage-sensitive and disease-related genes ( Table 1 ). These insights can be applied to predict the pathogenicity of CNVs and have great potential for accelerating the understanding of CNVs in disease. We propose that investigating CNV of genes in ORRs is an efficient mechanism to identify pathogenic CNVs. Classification of human genes We obtained 20,907 human protein-coding genes from Ensembl release 52 (hg18) [49] . We used 7,294 ohnologs and 9,027 small-scale duplicated genes (blastp: e<10 −7 and alignment >30%) from Makino and McLysaght [25] and ( Supplementary Data 1 ). We defined 6,064 genes that were neither ohnologs nor small-scale duplicated genes as singletons. Dosage-sensitive singletons We conducted an all-against-all blastp search for protein sequences for each of chimpanzee, macaque, mouse, rat, dog, cow, opossum and chicken, and got duplicated genes (e<10 −7 and alignment >30%) and singletons (others) for each vertebrate. We identified single-copy orthologous groups, which have not experienced gene duplication in human, chimpanzee, macaque, mouse, rat, dog, cow, opossum and chicken using one-to-one orthologous relationships between human and the vertebrate singletons from Ensembl release 52. Of the human singletons, 1,151 were singletons in all genomes analysed and we designated these human dosage-sensitive singletons. Genomic locations and human orthologs We obtained gene locations for human and eight vertebrates (chimpanzee, macaque, mouse, rat, dog, cow, opossum and chicken) and their orthology from Ensembl release 52. Genomic locations of centromere and telomere for the vertebrates were derived from UCSC ( http://genome.ucsc.edu ). Genes with CNVs We downloaded CNVs in the human genome from the Database of Genomic Variants version 9 ( http://projects.tcag.ca/variation ). We classified the CNVs in three categories giving 18,102 short (<3 kb), 16,121 medium (3–10 kb) and 24,456 long CNVs (≥10 kb). When the entire coding-sequence of a gene is within one of the CNVs, we defined the gene as a CNV gene. We identified 6,711 CNV genes ( Supplementary Data 1 ). We obtained CNVs in seven vertebrate species from the literature (chimpanzee [8] , macaque [7] , mouse [6] , rat [5] , dog [4] , cow [3] and chicken [2] ). According to the genomic location of their CNVs, 1,006, 78, 445, 306, 329, 251 and 365 genes displayed CNVs for chimpanzee, macaque, mouse, rat, dog, cow and chicken, respectively. Segmental duplications We obtained 9,913 intragenic SDs (>5 kb and >90% identity) from Cheung et al. [44] Genomic locations for the SDs based on human genome assembly hg17 were converted to those based on hg18 by liftOver ( http://genome.ucsc.edu/cgi-bin/hgLiftOver ). Syntenic genes between human and chicken We obtained orthologous gene pairs between human and chicken from Ensembl release 52. We used orthologous gene pairs located within 10 genes for each genome in order to find gene order conserved regions between human and chicken, resulting in that we identified 687 syntenic blocks in the human genome. Thus, we got 10,979 human syntenic genes in the syntenic regions between human and chicken. Protein complex genes We obtained 2,708 genes encoding subunits of protein complexes from Human Protein Reference Database release 9 [50] , in which 1,192 and 1,516 protein complex genes are ohnologs and non-ohnologs, respectively. Disease genes We obtained 2,548 disease genes from ‘Morbidmap’ produced by Online Mendelian Inheritance in Man ( ftp://ftp.ncbi.nih.gov/repository/OMIM/morbidmap ), in which 1,201 and 1,347 disease genes are ohnologs and non-ohnologs, respectively. How to cite this article: Makino, T. et al. Genome-wide deserts for copy number variation in vertebrates. Nat. Commun. 4:2283 doi: 10.1038/ncomms3283 (2013).